Room temperature near unity spin polarization in 2D Van der Waals heterostructures The generation and manipulation of spin polarization at room temperature are essential for 2D van der Waals (vdW) materials-based spin-photonic and spintronic applications. However, most of the high degree polarization is achieved at cryogenic temperatures, where the spin-valley polarization lifetime is increased. Here, we report on room temperature high-spin polarization in 2D layers by reducing its carrier lifetime via the construction of vdW heterostructures. A near unity degree of polarization is observed in PbI 2 layers with the formation of type-I and type-II band aligned vdW heterostructures with monolayer WS 2 and WSe 2 . We demonstrate that the spin polarization is related to the carrier lifetime and can be manipulated by the layer thickness, temperature, and excitation wavelength. We further elucidate the carrier dynamics and measure the polarization lifetime in these heterostructures. Our work provides a promising approach to achieve room temperature high-spin polarizations, which contribute to spin-photonics applications. Van der Waals (vdW) heterostructures formed by different two-dimensional (2D) materials are emerging as an excellent platform for both fundamental research and technical applications [1] , [2] , [3] , due to the unique photonic, optoelectronic properties of the individual materials, and the combination their advantages in heterostructures [4] , [5] , [6] , [7] . The band alignment at the interface of the vdW heterostructures can modulate the interfacial carrier behaviors, which is essential for device applications [8] . Up to now, vdW heterostructure-based logic transistors [9] , modulators [10] , light-emitting diodes (LEDs) [11] , fast photodetectors [12] , and photovoltaic cells [13] have been realized, which make them important building blocks for photonic and optoelectronic devices and integrated circuits. With the development of quantum information science, the 2D materials-based spin-photonic devices are highly desirable. The generation and control of spin polarization is at the heart of this field. One recent progress along this direction is the light-induced spin and valley polarization in transition metal dichalcogenides (TMDCs) [14] , [15] , [16] , [17] and their heterostructures [18] , [19] , [20] , [21] , [22] . However, most of these studies were performed at low temperature with high-quality samples, so as to reduce the intervalley scattering and increase the spin-valley polarization lifetime [23] , [24] . It is therefore greatly desirable to find new materials and/or mechanism to obtain a high degree of spin polarization at room temperature, which is essential for practical spintronic applications. Compared to typical TMDCs such as WS 2 and WSe 2 , layered lead iodine (PbI 2 ) has a wider bandgap and higher light absorption coefficient, showing potential optoelectronic applications [25] , [26] , [27] , [28] , such as photodetectors [29] , [30] , [31] , [32] , X-ray or γ-ray detection [33] , [34] , and optically pumped lasers [35] . PbI 2 has a hexagonal crystal pattern composed of covalently bonded repeating sequences of I-Pb-I atomic layers, with weak vdW interaction between the two layers [25] , [26] . The bandgap can be tuned from a direct gap of 2.28 eV to an indirect-gap of 2.63 eV when reducing its thickness or a fine-tuning by applying strain [25] , [26] . Due to the vdW nature, layered PbI 2 can easily form heterostructures with other TMDCs materials [36] , exhibiting versatile band alignment [37] , [38] . Furthermore, since PbI 2 can be used as a precursor of lead halide perovskite, the conversion from PbI 2 /TMDCs to perovskite/TMDCs heterostructures have been realized [39] , [40] , which further extends the applications of PbI 2 . The formation of high-quality heterostructures provides the opportunity to manipulate the carrier dynamics in the vertical direction and affects the carrier lifetime [41] . Here, we report on room temperature high-spin polarization in PbI 2 layers via the construction of heterostructures with monolayer TMDCs. Due to the reduction of carrier lifetime, a near-unity degree of polarization at room temperature is observed from both layered PbI 2 /monolayer-WS 2 type-I and PbI 2 /monolayer-WSe 2 type-II band aligned heterostructures. The spin polarization related to the carrier lifetime can be manipulated by the material thickness, temperature, and excitation wavelength, providing versatile control means for further practical applications. In addition, we investigate the polarized carrier dynamics in heterostructures and reveal the polarization lifetime by time-resolved polarization experiments. This work not only provides a basis for controlling carrier dynamics and spin polarization in 2D vdW heterostructures but also offers a strategy to achieve a high degree of spin polarization at room temperature, promising for spin-photonics applications. PbI 2 /WS 2 heterostructures and near-unity polarization The heterostructures consisting of a bottom WS 2 monolayer and top PbI 2 layers with different thicknesses were prepared with a two-step physical vapor deposition (PVD) method. Typical heterostructures show a triangular shape with a uniform and smooth surface (Fig. 1a ). Based on the calculated electronic structures from previous works [38] , [41] , the formed PbI 2 /WS 2 heterostructures show a type-I band alignment, such that the photogenerated electrons and holes can be transferred from the PbI 2 to the WS 2 monolayer (Fig. 1a ), which is also confirmed by our experimental results. Since circularly polarized photons carry angular momentum components, the absorption of a circularly polarized laser leads to the so-called optical spin injection to the materials [42] . 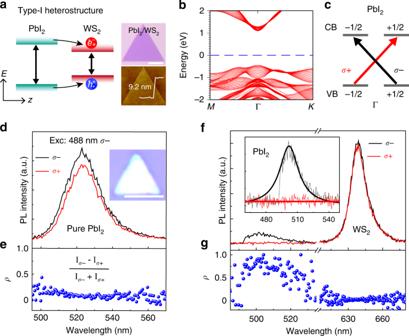Fig. 1: Spin polarization mechanism and spectrum of PbI2/WS2heterostructures. aSchematic of the type-I heterostructure for the study of the carrier interlayer transportation. Both electrons and holes transfer from PbI2to WS2. The images on the right are optical and AFM micrographs of a PbI2/WS2heterostructure with a thickness of 9.2 nm.bBand structure for the PbI2thin film with a thickness of 20 layers, which is spin degenerate.cSchematic illustration of the polarized optical transitions in PbI2thin films.dCircularly polarized PL spectra from pure PbI2at room temperature.eCorresponding degree of polarizationρof pure PbI2PL calculated from the PL spectra shown in figure (d).fCircularly polarized PL spectra of a representative PbI2/WS2heterostructure at room temperature.gCorresponding degree of polarizationρcalculated from the PL spectra shown in figure (f). All length of the scale bar is 10 µm. Figure 1b shows the band structure for the PbI 2 thin film with a thickness of 20 layers (details of density-functional theory calculations are given in Supplementary Note 1 ). Both the valence band maximum (VBM) and conduction band minimum (CBM) locate at the Г point and are spin degenerate because the thin film has the inversion symmetry and time-reversal symmetry. Figure 1c shows schematically the optical selection rules for PbI 2 layers at Γ point. The right-handed (σ+) polarized photon carrying an angular monument of \(+ \hbar\) causes the transition from the spin state −1/2 to +1/2, while left-handed (σ−) excitation referring to the transition from the spin state +1/2 to −1/2. The degree of photoluminescence (PL) circular polarization ( ρ ) can be defined as ρ PL = ( Ι σ − / σ + − Ι σ +/ σ − )/( Ι σ + + Ι σ − ) under σ−/σ+ polarized excitation, where Ι σ + and Ι σ − denote the σ+ and σ− polarized PL intensities, respectively. Fig. 1: Spin polarization mechanism and spectrum of PbI 2 /WS 2 heterostructures. a Schematic of the type-I heterostructure for the study of the carrier interlayer transportation. Both electrons and holes transfer from PbI 2 to WS 2 . The images on the right are optical and AFM micrographs of a PbI 2 /WS 2 heterostructure with a thickness of 9.2 nm. b Band structure for the PbI 2 thin film with a thickness of 20 layers, which is spin degenerate. c Schematic illustration of the polarized optical transitions in PbI 2 thin films. d Circularly polarized PL spectra from pure PbI 2 at room temperature. e Corresponding degree of polarization ρ of pure PbI 2 PL calculated from the PL spectra shown in figure ( d ). f Circularly polarized PL spectra of a representative PbI 2 /WS 2 heterostructure at room temperature. g Corresponding degree of polarization ρ calculated from the PL spectra shown in figure ( f ). All length of the scale bar is 10 µm. Full size image Experimentally observed polarized PL spectra (Fig. 1d ) and the calculated ρ (Fig. 1e ) from pure PbI 2 layers (grown on SiO 2 /Si substrate, about 100 nm) show a small ( ρ ≈ 0.1 for 488 nm excitation) degree of polarization and also an excitation wavelength dependence that further away from the resonance excitation leads to a much smaller value (Supplementary Fig. 5 ). Such a low polarization can be due to the spin relaxation during the carrier lifetime. Considering the carrier lifetime ( τ c ) and spin relaxation time ( τ s ), the measured degree of the polarization can be expressed as P = P 0 /(1 + τ c / τ s ), where P 0 is the polarization without spin relaxation [42] . For carrier lifetimes much longer than the spin relaxation ( τ c » τ s ), the polarization will be small. In order to obtain a high polarization of P , one should either increase the spin relaxation time ( τ s ) or decrease the carrier lifetime ( τ c ). Although the former depends on the detailed material and experiment conditions and thus is hard to control, the latter can be engineered by stacking different 2D materials to form a vdW heterostructure. The mechanism behind is that in a vdW heterostructure the band alignment leads to interlayer charge transfer that would significantly reduce the carrier lifetime and thus increase the spin polarization. For pure WS 2 monolayer, the circular polarization excitation creates the valley polarization and the degree of polarization is in general small under off-resonance excitation at room temperature (Supplementary Fig. 6 ) [43] . The PbI 2 /WS 2 heterostructures were excited with σ− excitation and the PL emission with σ+ and σ− polarizations were detected (Fig. 1f ). For the PL signal from PbI 2 , we observe that the dominating emission is σ− polarized (black). Compared to the pure PbI 2 layers, the degreed of polarization of PbI 2 in heterostructures increases dramatically, almost reaching 100% at room temperature (Fig. 1g ), consistent with our above mechanism. Explicitly, the carrier transfer process dramatically reduces the carrier lifetime of PbI 2 [41] , which leads to a small value of τ c / τ s hence resulting in near-unity spin polarizations under resonance excitation. In contrast, the degree of polarization of the WS 2 monolayer in heterostructures decreases, showing almost no polarization. Therefore, vdW heterostructures, where extra decay channels reduce the carrier lifetime largely, provide an excellent platform to achieve a high degree of polarization. To further verify the carrier lifetime enhanced the degree of polarization, we investigated how it depends on the thickness of the PbI 2 layer while maintaining the bottom monolayer WS 2 in the heterostructures. For pure PbI 2 layers with different thicknesses, the PL shows similar decay curves in time-resolved PL (TRPL) spectra (Supplementary Fig. 7 ). In contrast, increasing the thickness of the PbI 2 layer in heterostructures will increase its carrier lifetime, which would decrease the obtained polarization. 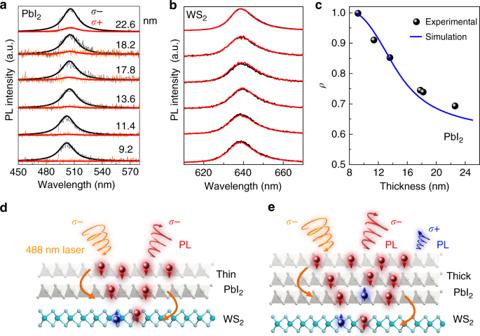Fig. 2: Thickness-dependent spin polarization and the underlying mechanism in PbI2/WS2heterostructures. a,bCircularly polarized PL spectra of PbI2and WS2in PbI2/WS2heterostructures with different thicknesses.cDegree of polarizationρof PbI2as a function of thickness of the heterostructures. The solid line represents the numerical simulation result.d,eSchematic illustrations of the resulting spin polarization in the thin and thick PbI2/WS2heterostructures. The curled curves represent the incident light and the PL emissions. The red balls represent spin-down electrons, and the blue balls represent spin-up electrons. Figure 2 displays the circularly polarized PL spectra from PbI 2 /WS 2 heterostructures with the total thickness varying from 9.2 to 22.6 nm, with σ− excitation. For the PL signal from PbI 2 (Fig. 2a ), besides the overall dominating emission with σ− polarization (black), we observe that the weak emission signal from the σ+ polarization (red) increases with the increasing thickness of heterostructures. In contrast, the relative intensities of σ+ and σ− emission from the monolayer WS 2 in the heterostructures are almost unchanged (Fig. 2b ), showing the small degree of polarization as we discussed previously. With the spectra in Fig. 2a , we have calculated ρ for the PbI 2 PL from different heterostructures and show that ρ decreases from 0.998 to 0.693 as the heterostructures thickness increases from 9.2 to 22.6 nm (Fig. 2c ). Fig. 2: Thickness-dependent spin polarization and the underlying mechanism in PbI 2 /WS 2 heterostructures. a , b Circularly polarized PL spectra of PbI 2 and WS 2 in PbI 2 /WS 2 heterostructures with different thicknesses. c Degree of polarization ρ of PbI 2 as a function of thickness of the heterostructures. The solid line represents the numerical simulation result. d , e Schematic illustrations of the resulting spin polarization in the thin and thick PbI 2 /WS 2 heterostructures. The curled curves represent the incident light and the PL emissions. The red balls represent spin-down electrons, and the blue balls represent spin-up electrons. Full size image This phenomenon is related to the changing of carrier lifetime and can be understood by following the equation P ( X ) = P 0 /(1 + τ eff( X ) / τ s ), where τ eff is the effective lifetime of the carriers, X is the thickness of the PbI 2 layers (Supplementary Note 2 ). Based on the coupled rate equations of spin injected carriers, we performed simulations of the degree of polarization for PbI 2 PL in heterostructures (solid line in Fig. 2c ) as a function of heterostructure thickness. One can see that the simulations are in good agreement with our experimental data (solid spheres in Fig. 2c ). We illustrate the phenomena in Fig. 2d, e for typical thin and thicker PbI 2 in heterostructures that the spin-flip within the longer carrier lifetime leads to a smaller degree of polarization. We also measured excitation power dependent circularly polarized PL spectra, and reveal only a slight decrease of the ρ of PbI 2 PL when the excitation power increases from 2 to 10 μW (Supplementary Fig. 8 ). Polarization dynamics To probe the polarization lifetime, we have excited a 13.6 nm thick PbI 2 /WS 2 heterostructure with σ+ polarized 100-fs laser at 441 nm, and recorded the spectrally integrated and time-resolved σ+ and σ− PL emission, respectively. 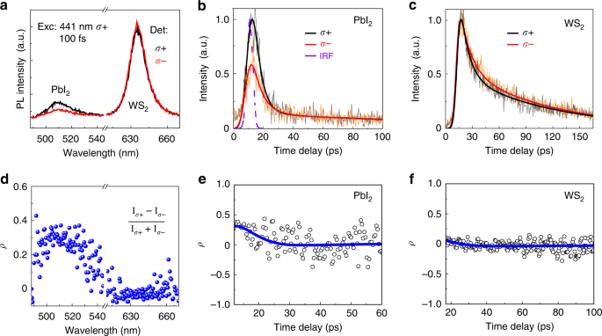Fig. 3: Spin polarization dynamics of PbI2/WS2heterostructures. a–cCircularly polarized PL spectra (a) and TRPL data from PbI2(b), and WS2(c) of PbI2/WS2heterostructures.d–fCorresponding degree of polarizationρas a function of wavelength and time calculated from the PL and TRPL spectra. For excitation, a 441 nmσ+ polarized fs-pulsed laser beam was used. The integrated PL intensity (Fig. 3a ) shows a degree of polarization of about 0.3 for PbI 2 , and almost zero degree of polarization for WS 2 (Fig. 3c ). Compared with the experiments under the excitation at 488 nm, we observed a reduced degree of polarization due to the off-resonance excitation, which is similar to the observations of many TMDCs atomic layers under different excitation photon energies [14] , [44] . Almost no polarization can be observed for the same heterostructures exited with 100 fs-pulsed laser at 400 nm, since they are even further off-resonance (Supplementary Fig. 9 ). In Fig. 3b , we show the σ+ (black) and σ− (red) PbI 2 PL emission decay detected in the spectral range from 2.30 to 2.53 eV by a streak camera. The dashed line represents the instrument response function (IRF) obtained from pure laser pulses under the same experimental condition. After the deconvolution of the measured decay curves from the IRF and the fitting, we obtain the decay times for the σ+ and σ− polarized PbI 2 PL emission, which are 15.7 and 27.5 ps, respectively. With these two time-resolved polarized PL decays, we can calculate the degree of polarization as a function of time, revealing the polarization lifetime of about 15 ps (Fig. 3e ). For resonance excitation, the polarization lifetime is expected to be longer [45] , which could lead to a higher degree of polarization due to a smaller τ c / τ s . For the WS 2 monolayer in the heterostructures, the σ+ and σ− polarized PL emissions show similar decay curves of about 49 ps (Fig. 3c ), consistent with the integrated PL spectra, leading to the non-observable polarization lifetime (Fig. 3f ). It should be noted that the dominating excited carriers account for the WS 2 PL in heterostructures originate from the transferred carriers, not the optical valley initialization in pure WS 2 monolayer. Fig. 3: Spin polarization dynamics of PbI 2 /WS 2 heterostructures. a – c Circularly polarized PL spectra ( a ) and TRPL data from PbI 2 ( b ), and WS 2 ( c ) of PbI 2 /WS 2 heterostructures. d – f Corresponding degree of polarization ρ as a function of wavelength and time calculated from the PL and TRPL spectra. For excitation, a 441 nm σ + polarized fs-pulsed laser beam was used. 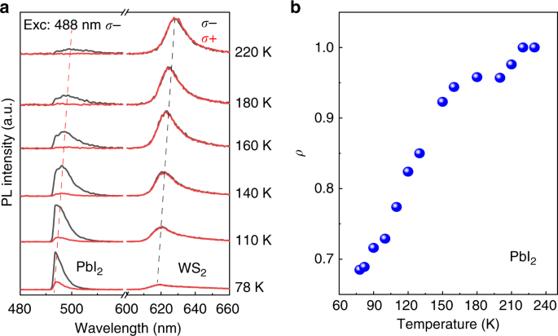Fig. 4: Temperature-dependent degree of polarization from PbI2/WS2heterostructures. aCircularly polarized PL spectra of PbI2/WS2heterostructure at different temperatures for excitation with a 488 nmσ− polarized CW laser beam.bDegree of polarizationρof PL from PbI2as a function of temperature, showing a decreasing tendency at lower temperatures. Full size image Temperature-dependent polarization Figure 4a shows the temperature-dependent circularly polarized PL spectra of PbI 2 /WS 2 heterostructures. With decreasing temperature, the PL emission from PbI 2 and WS 2 blue shifts, as indicated by the dashed line. The PL intensity of PbI 2 largely increases in comparison with that of WS 2 . This is because the interlayer charge transfer from PbI 2 to WS 2 is momentum mismatched. This process is only allowed with the assistance of phonons, which is suppressed greatly at low temperatures. As a result, the carrier lifetime in the PbI 2 layer is increased with a decrease in temperature, similar to the effect of increasing layer thickness, which leads to a decrease in the degree of polarization ρ . Indeed, we found ρ of PbI 2 PL in heterostructures decreases from 0.99 to 0.68 when the temperature decreases from 220 to 78 K (Fig. 4b ). This temperature dependence is in contrast to the case for the pure TMDCs, where the degree of polarization in TMDCs monolayer normally increases at lower temperatures due to the reduced intervalley scattering. In control measurements with pure PbI 2 layers, we find that the small ρ at room temperature slightly increases at low temperatures (Supplementary Fig. 11 ), which indicates that the observed temperature-dependent polarization in heterostructures does not originate from the intrinsic property of pure PbI 2 but due to interlayer charge transfer process. Our results suggest that PbI 2 in PbI 2 /WS 2 heterostructures shows a higher polarization at room temperature, which makes them even more practical for device applications. Fig. 4: Temperature-dependent degree of polarization from PbI 2 /WS 2 heterostructures. a Circularly polarized PL spectra of PbI 2 /WS 2 heterostructure at different temperatures for excitation with a 488 nm σ − polarized CW laser beam. b Degree of polarization ρ of PL from PbI 2 as a function of temperature, showing a decreasing tendency at lower temperatures. Full size image Near-unity polarization from PbI 2 /WSe 2 heterostructures We have studied the degree of polarization in the PL spectra emitted from PbI 2 /WSe 2 heterostructures, which have the type-II band alignment that photogenerated electrons can transfer from WSe 2 to PbI 2 and holes transfer from PbI 2 to WSe 2 (Fig. 5a ). The formation of type-II alignment also reduces the carrier lifetime in PbI 2 , due to the extra decay channel [38] . Therefore, a high degree of polarization is expected for PbI 2 PL in PbI 2 /WSe 2 . 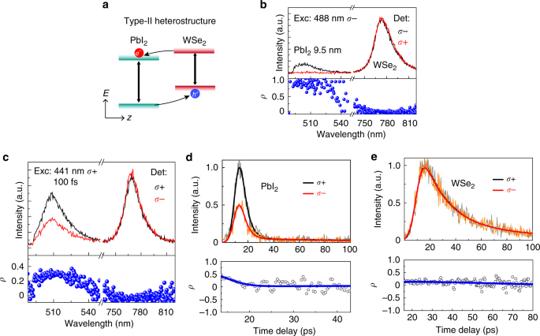Fig. 5: Degree of spin polarization and the dynamics in PbI2/WSe2heterostructures. aSchematic of the type-II band alignment and the corresponding photogenerated carrier behaviors in PbI2/WSe2heterostructures.bCircularly polarized PL spectra from a 9.5 nm thick PbI2/WSe2heterostructure, and the corresponding calculatedρas a function of wavelength. The excitation is 488 nmσ− polarized CW laser.c–eCircularly polarized PL spectra (c) and TRPL data from PbI2(d) and WSe2(e) in PbI2/WSe2heterostructure, and the corresponding degree of polarizationρcalculated from PL and TRPL spectra. Excitation with 441 nmσ+ polarization femtosecond laser pulses. Figure 5b shows the circular polarization-resolved PL emission of a 9.5-nm-thick heterostructure, under σ− polarized continuous-wave (CW) laser excitation at 488 nm. For PbI 2 PL emission, we observe that σ− polarization (black) dominates the whole emission. The calculated degree of polarization (Fig. 5b , lower panel) approaches 100% at room temperature, which is due to the largely reduced carrier lifetime with a very small τ c / τ s . Similar to PbI 2 /WS 2 heterostructures, the thicker heterostructures show a slightly smaller polarization value (Supplementary Fig. 12 ). The valley polarization of WSe 2 is very low because the excitation light is far from resonance, even though its carrier lifetime reduces as well. We further performed time-resolved σ+ and σ− polarized PL emission experiments under the excitation of σ+ polarized 100-fs laser at 441 nm. The integrated PL intensity shows a degree of polarization of about 0.3 for PbI 2 , and almost zero degree of polarization for WSe 2 (Fig. 5c ). After the deconvolution of the measured decay curve from the IRF and the fitting (Fig. 5d ), we obtain the σ+ and σ− polarized PL emission with 7.5 and 9.44 ps lifetime, and the polarization lifetime of 13 ps in the PbI 2 /WSe 2 heterostructure. Considering the smaller value of P 0 under non-resonance excitation, the obtained τ c and τ s is general in agreement with the observed degree of polarization. For WSe 2, the σ+ and σ− polarized PL emissions show similar decay curves of about 30 ps (Fig. 5e ), showing a non-observable polarization lifetime, which agrees with the integrated PL spectra and the close to zero degree of polarization. With temperature-dependent polarization measurements, we find that the ρ of PbI 2 PL decreases with the temperature decreases (Supplementary Fig. 13 ), which is consistent with the temperature dependence in PbI 2 /WS 2 heterostructure. Fig. 5: Degree of spin polarization and the dynamics in PbI 2 /WSe 2 heterostructures. a Schematic of the type-II band alignment and the corresponding photogenerated carrier behaviors in PbI 2 /WSe 2 heterostructures. b Circularly polarized PL spectra from a 9.5 nm thick PbI 2 /WSe 2 heterostructure, and the corresponding calculated ρ as a function of wavelength. The excitation is 488 nm σ − polarized CW laser. c – e Circularly polarized PL spectra ( c ) and TRPL data from PbI 2 ( d ) and WSe 2 ( e ) in PbI 2 /WSe 2 heterostructure, and the corresponding degree of polarization ρ calculated from PL and TRPL spectra. Excitation with 441 nm σ + polarization femtosecond laser pulses. Full size image In conclusion, we have demonstrated the realization of a near-unity spin polarization in layered PbI 2 /WS 2 and PbI 2 /WSe 2 in vdW heterostructures at room temperature via vdW engineering. The underlying physics relies on the reduction of the carrier lifetime through interlayer carrier transfer in vdW heterostructures. We observe a thickness-dependent degree of polarization of PbI 2 in PbI 2 /WS 2 heterostructures, that the thicker the PbI 2 layers the smaller the degree of polarization. By time-resolved circulary polarization measurements, we reveal the spin polarization lifetime of PbI 2 in heterostructures. The degree of polarization is also found to have an excitation power and wavelength dependence. The higher the excitation power leads to a slight decrease in the polarization. For excitations with photon energy away from the resonance, we observed a smaller polarization. The polarization decreases to zero under the excitation of 400 nm laser. Furthermore, we also demonstrated that the near-unity degree of polarization can be obtained in a PbI 2 and monolayer-WSe 2 heterostructure with a type-II band alignment, which can also be understood by manipulating the carrier lifetime. The realization of high-spin polarization via the formation of heterostructure in principle can be applied with other substrates that quenches the PL. However, one needs to consider the balance between the increasing degree of polarization and the PL quenching. For PbI 2 /TMDCs heterostructures, the PL in PbI 2 is quenched about one order of magnitude but the remaining intensity is still comparable with that of typical monolayer TMDCs. On the other hand, monolayer TMDCs provide an excellent platform to construct a high-quality heterostructure with PbI 2 through vdW interaction, facilitates the efficient transport of carriers. Moreover, for future applications, not only the high-spin polarization, but also spin coherence are of great importance. The detailed study of the spin coherence should take into account the effect of the temperature-related dephasing and is an interesting topic for future study. Our study provides a promising strategy via vdW engineering to achieve a high degree of polarization in vdW 2D materials at room temperature, which could provide valuable information for spintronics. Sample preparation The PbI 2 /TMDCs heterostructures were synthesized by a two-step PVD method. Briefly, monolayer TMDCs (WS 2 , WSe 2 ) serving as the bottom layers for the heterostructures were synthesized first by PVD method. In the second step, lead iodide powder was placed in the central area of the tube furnace, the substrates with grown monolayer TMDCs from the first step were placed in the downstream area of the tube furnace. The pressure in the furnace was drawn to 40 mtorr by a vacuum pump and the argon flow rate was maintained at 20 sccm. The heating lasts 10 min at a temperature of 400 °C. By varying the deposition temperature of PbI 2 from 180 to 220 °C, we obtained a growth trend of thin to thick PbI 2 /TMDCs heterostructures. The thicknesses of the heterostructures were measured with an atomic force microscope (AFM). By the same experimental method, pure PbI 2 layers can be grown on SiO 2 /Si or mica substrates. In order to improve the environmental stability of the prepared PbI 2 /WS 2 and PbI 2 /WSe 2 heterostructures in optical measurement, all samples were encapsulated with polydimethylsiloxane (PDMS). Steady-state circular polarization-resolved PL spectroscopy Steady-state circular polarization-resolved PL measurements were conducted using a confocal microscope (WITec, alpha-300) equipped with a ×50 objective (Zeiss, 0.75 NA). To create the circularly polarized excitation light source, the laser beam first passes through a linear polarizer (GTH10M-AM-A, Thorlabs), and then a quarter-wave plate (AQWP05M-600, Thorlabs). The circularly polarized beam is reflected by a cube beam splitter (CCM1-BS013/M, Thorlabs) and focused on the sample. The signal is collected by the same objective and is detected by a spectrometer (UHTS300) after passing through a razor edge long pass 488 nm laser filter, a quarter-wave plate and a polarizer (WP25M-UB, Thorlabs). Left-handed and right-handed PL components of the signal are distinguished by rotating the polarizer. Continuous-wave Ar ion laser (Coherent, Sapphire LP) at 488 nm (excitation power of 2 μW) is normally used as the excitation source. For comparison, 400 nm and 441 nm fs lasers pulses (excitation power of about 20 μW) were used as well. During the experiment, 150 grooves/mm gratings were used for PL measurements. Low temperature circular polarization-resolved PL measurement The circularly polarized light is focused by a long working distance objective lens (×50, Zeiss, NA 0.55) onto the sample located in the cryostat (ST-500, Janis Research Company). The method of circular polarization-resolved PL measurement is the same as that at room temperature. Dynamics of circular polarization-resolved PL The dynamics of circular polarization-resolved PL of heterostructures were measured using the same optical microscope (WITec, alpha-300) equipped with a streak camera (C10910, Hamamatsu). A mode-locked Ti: sapphire laser (Tsunami 3941-X1BB, Spectral Physics) (pulse width 100 fs, repetition rate 80 MHz) was used as the fundamental excitation source. Photons at 400 and 441 nm were generated via the frequency doubling from the fundamental 800 and 882 nm with a BBO crystal. The same optical paths were used to generate circularly polarized 400 and 441 nm excitation beams. The left- and right-handed circular polarization PL were guided into the streak camera for time-resolved measurements, which were distinguished by the same optical system described for the steady-state measurements.